A nanostructured cathode architecture for low charge overpotential in lithium-oxygen batteries The lithium-oxygen battery, of much interest because of its very high-energy density, presents many challenges, one of which is a high-charge overpotential that results in large inefficiencies. Here we report a cathode architecture based on nanoscale components that results in a dramatic reduction in charge overpotential to ~0.2 V. The cathode utilizes atomic layer deposition of palladium nanoparticles on a carbon surface with an alumina coating for passivation of carbon defect sites. The low charge potential is enabled by the combination of palladium nanoparticles attached to the carbon cathode surface, a nanocrystalline form of lithium peroxide with grain boundaries, and the alumina coating preventing electrolyte decomposition on carbon. High-resolution transmission electron microscopy provides evidence for the nanocrystalline form of lithium peroxide. The new cathode material architecture provides the basis for future development of lithium-oxygen cathode materials that can be used to improve the efficiency and to extend cycle life. The Li-O 2 battery is currently the subject of much scientific investigation because of its potential for very high-energy density exceeding that of any other existing energy storage systems [1] , [2] . In the Li-O 2 battery, a porous oxygen cathode is used to store the solid products generated from the reaction of Li cations with O 2 during discharge. The cathode may contain a catalyst in some form to promote the discharge reaction. It has been found that a variety of factors dictate the nature of electrochemical reactions in Li-air cells including the nature of the catalyst, the catalyst distribution on the porous cathode, the pore volume of the cathode and the type of organic electrolyte used [3] , [4] , [5] , [6] , [7] , [8] , [9] , [10] . One of the major challenges for the development of Li-O 2 batteries is to lower the high overpotential during charge. A large overpotential on charge, even at very low current densities, can result in a very low round-trip efficiency (<60%), low power capability and poor cycle life. Various electrocatalysts including carbons, metals and metal oxides have been examined as the cathode catalysts in the Li-O 2 cells to lower the charge overpotential. Some of the early work on Li-O 2 batteries was based on carbonate electrolytes including catalysts such as α-MnO 2 , Co 3 O 4 , Mn 3 O 4 and PtAu [11] , [12] , [13] , [14] , [15] . However, carbonate electrolytes were found to decompose in Li-O 2 batteries [1] , [16] , [17] and consequently researchers turned to ether-based electrolytes, which have greater stability [8] , [11] , [18] . In a dimethoxyethane-based electrolyte, McCloskey et al. [19] investigated the electrocatalytic role of Au, Pt and MnO 2 nanoparticles and found that none of these nanoparticles performs better than just a carbon surface. They also found that the charge potential at the beginning of the charge cycle is low (~3.4 V) but rises to above 4 V during the first cycle. Nazar et al. [20] investigated the use of small cobalt oxide nanoparticles and obtained a decrease in the charge potential to ~3.8 V from ~4.2 V, which they attributed to mass transport effects rather than conventional electrocatalytic effects of the particles. There may be a number of other contributing factors for the large charge overpotentials other than the lack of an effective electrocatalyst. Poor electronic conductivity of Li 2 O 2 discharge product may limit the charge process, which depends on electron transport to the Li 2 O 2 /electrolyte interface [21] , [22] , [23] . Contaminants in the Li 2 O 2 discharge product from electrolyte decomposition such as Li 2 CO 3 may also cause a higher charge potential. McCloskey et al. [24] showed that decomposition may result from reaction of the electrolyte with defects on the carbon surface, whereas Bruce et al. [25] showed that oxidation of the carbon surface can occur at voltages as low as 3.5 V during charge in the presence of Li 2 O 2 . Interestingly, Norskov et al. [26] have shown that the theoretical overcharge potential for a Li 2 O 2 film is only 0.2 V for some surfaces, assuming no limitations in charge transport through Li 2 O 2 to the Li 2 O 2 -electrolyte interface. Therefore, it may be possible to significantly lower the charge potential if solutions to the above problems can be discovered. In this paper, we describe a conceptually new approach as illustrated in Fig. 1 based on a new cathode architecture for the Li-O 2 cells that shows promising results for solving the charge overpotential problem. The cathode architecture addresses the electrolyte decomposition problem with a porous carbon passivated by a protective Al 2 O 3 coating applied by atomic layer deposition (ALD). Very small Pd nanoparticles attached to the surface by ALD act as effective electrocatalysts and seem to promote formation of a nanocrystalline form of Li 2 O 2 that provides good electronic transport. The resulting low charge overpotential is about 0.2 V. The lithium peroxide is characterized by X-ray diffraction (XRD), scanning electron microscopy (SEM) as well as high-resolution transmission electron microscopy (HRTEM) techniques. Computational modelling is used to provide an insight into the role of the Al 2 O 3 protective coating and the Pd nanoparticles for preventing electrolyte decomposition and catalysing the lithium peroxide decomposition, respectively. 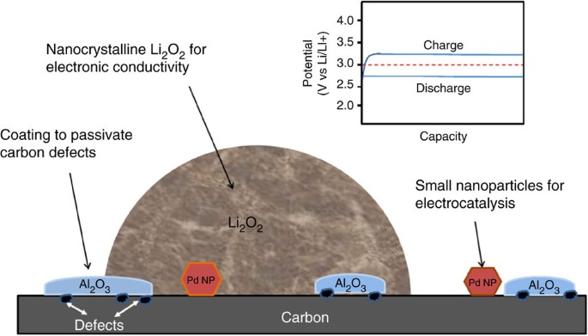Figure 1: Schematic of the nanostructured cathode architecture. This figure shows the Al2O3coating, the palladium nanoparticles and the nanocrystalline lithium peroxide, all of which contribute to lowering the overpotential. The inset shows a hypothetical charge/discharge voltage profile versus capacity. Figure 1: Schematic of the nanostructured cathode architecture. This figure shows the Al 2 O 3 coating, the palladium nanoparticles and the nanocrystalline lithium peroxide, all of which contribute to lowering the overpotential. The inset shows a hypothetical charge/discharge voltage profile versus capacity. Full size image Synthesis and characterization of the cathode architecture The synthesis of the new cathode architecture was done using ALD, a technique for preparing thin films that employs self-limiting chemical reactions between gaseous precursors and a solid surface allowing atomic scale control over the film thickness and composition [27] . One of the distinguishing attributes of ALD is the capability to deposit coatings on surfaces with complex topographies and to infiltrate mesoporous materials, important for the Al 2 O 3 coatings used for the cathode in this study [28] , [29] , [30] . The ALD technique can also be used to synthesize supported noble metal catalysts, such as Pd used in this work, in the size range from subnanometres to nanometres [31] , [32] , [33] , [34] . Super P Li (SPL) conductive carbon black with a typical particle size of 40 nm and a surface area of 62 m 2 g −1 was used as the catalyst support material. We first coated the carbon surface with three cycles of Al 2 O 3 by ALD, which deposits on the carbon defect sites [35] , [36] and thus acts to passivate the defects on the carbon surface ( Supplementary Note 1 ). Then, three cycles of ALD were used to load palladium nanoparticles on the surface to serve as electrocatalytic sites. Representative HRTEM images of the uncoated carbon, Al 2 O 3 -coated carbon and Al 2 O 3 -coated carbon with Pd nanoparticles are shown in Fig. 2 . The pristine carbon surface is shown in Fig. 2a . In Fig. 2b , it is shown that the carbon surface is only partially covered by the Al 2 O 3 after the three cycles of ALD. The partially covered carbon surface is characterized by islands of Al 2 O 3 that deposit on defect sites leaving some carbon surface exposed. The carbon defect sites could be, for example, carbonyl, alcohol and ether groups, which have been found to be reactive towards the tetramethylaluminium precursor in coating of polyethers [37] . The Al 2 O 3 islands are ~0.5 nm thick. 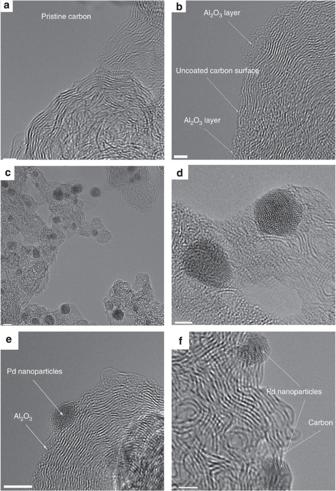Figure 2: HRTEM of the cathode structure. (a) Pristine super P carbon (scale bar, 2 nm); (b) carbon surface coated with three ALD cycles of Al2O3(Al2O3/C), (scale bar, 2 nm); (c–f) carbon+three ALD cycles Al2O3+Pd nanoparticles from three ALD cycles (Pd/C[Al2O3]), (scale bars in (c–f), 5 nm, 2 nm, 4 nm and 2 nm, respectively). Figure 2c,d shows the Pd nanoparticle size, size distribution and interparticle distance on the carbon support. Figure 2e,f shows that the Pd nanoparticles are attached to the carbon support as indicated by the wavy fringes characteristic of the carbon sheets. Moreover, the amorphous Al 2 O 3 islands are attached to regions of the carbon support surface near the Pd. The size of the Pd nanoparticles from the HRTEM images is in the range of 2–6 nm, although smaller Pd clusters cannot necessarily be ruled out. Figure 2: HRTEM of the cathode structure. ( a ) Pristine super P carbon (scale bar, 2 nm); ( b ) carbon surface coated with three ALD cycles of Al 2 O 3 (Al 2 O 3 /C), (scale bar, 2 nm); ( c – f ) carbon+three ALD cycles Al 2 O 3 +Pd nanoparticles from three ALD cycles (Pd/C[Al 2 O 3 ]), (scale bars in ( c – f ), 5 nm, 2 nm, 4 nm and 2 nm, respectively). Full size image The Pd nanoparticles and carbon surface were examined further using various spectroscopic techniques. X-ray adsorption spectroscopy (XAS) of the cathode in air at room temperature is shown in Fig. 3 along with the reference spectra recorded for Pd foil and PdO standard. X-ray absorption near-edge spectroscopy (XANES) are also given in Fig. 3 The XAS and XANES spectra indicate that the Pd nanoparticles from the three cycles of ALD are similar to bulk Pd, although the XANES spectra also shows that they are oxidized to some extent. The oxide fraction of the Pd nanoparticles is estimated to be about 20%, indicating that the Pd nanoparticle surface is largely oxidized. X-ray photoelectron spectroscopy (XPS) was used to investigate the nature of the Al 2 O 3 -coated carbon surface. The XPS spectra shown in Fig. 3 indicate that the Al 2 O 3 , coating by ALD, decreases the amount of defects on the carbon as evidenced by the disappearance of C=O ( Fig. 3c,d ) and O-H ( Fig. 3d ) peaks, although C-O bonds remain. 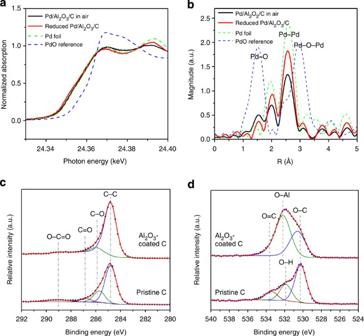Figure 3: XANES and XPS spectra. (a) XANES spectra for as-prepared 3c-Pd/3c-Al2O3/carbon in air and reduced 3c-Pd/3c-Al2O3/carbon along with spectra for metallic Pd foil reference and Pd oxide reference. (b) Fourier transform of X-ray absorption spectra (k2: Δk=2.8–11 Å−1) for as-prepared 3c-Pd/3c-Al2O3/carbon in air and reduced 3c-Pd/3c-Al2O3/carbon along with spectra for metallic Pd foil reference and Pd oxide reference. (c) C1s XPS spectra of uncoated and 3c-Al2O3-coated carbon, (d) O1s XPS spectra of uncoated and 3c-Al2O3-coated carbon. 3c represents three cycles of ALD. Figure 3: XANES and XPS spectra. ( a ) XANES spectra for as-prepared 3c-Pd/3c-Al 2 O 3 /carbon in air and reduced 3c-Pd/3c-Al 2 O 3 /carbon along with spectra for metallic Pd foil reference and Pd oxide reference. ( b ) Fourier transform of X-ray absorption spectra (k2: Δ k =2.8–11 Å −1 ) for as-prepared 3c-Pd/3c-Al 2 O 3 /carbon in air and reduced 3c-Pd/3c-Al 2 O 3 /carbon along with spectra for metallic Pd foil reference and Pd oxide reference. ( c ) C1s XPS spectra of uncoated and 3c-Al 2 O 3 -coated carbon, ( d ) O1s XPS spectra of uncoated and 3c-Al 2 O 3 -coated carbon. 3c represents three cycles of ALD. Full size image Performance of the cathode architecture The performance of this new cathode architecture as well as two architectures without Pd nanoparticles was then evaluated using a Swagelok-type cell [16] composed of a lithium metal anode, electrolyte (1 M LiCF 3 SO 3 in tetraethylene glycol dimethyl ether (TEGDME) impregnated into a glass fibre separator) and a porous cathode (13 mm diameter). 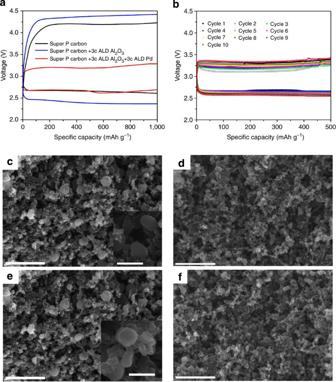Figure 4: Voltage profiles and SEM images. (a) Voltage profile during discharge-charge of cells (to 1,000 mAh g−1) based on super P carbon; super P carbon coated with Al2O3; and Al2O3-coated super P carbon further coated with Pd nanoparticles. The electrolyte used is TEGDME-LiCF3SO3; (b) voltage profile during discharge-charge of cells (to 5,00 mAh g−1) based on Al2O3-coated super P carbon further coated with Pd nanoparticles. The electrolyte used is TEGDME-LiCF3SO3. (c) SEM of 1st cycle after discharge to 500 mAh g−1(scale bar, 1 μm; scale bar of inset image, 400 nm); (d) SEM of 1st cycle after charge, (scale bar, 1 μm); (e) SEM of 10th cycle after discharge to 500 mAh g−1, (scale bar, 1 μm; scale bar of the inset image, 300 nm); (f) SEM of 10th cycle after charge, (scale bar, 1 μm). Figure 4 shows voltage profiles recorded during the first discharge/charge cycle obtained when a cell was subject to discharge first for the three cathode architectures: super P carbon only (C), super P coated with Al 2 O 3 (Al 2 O 3 /C), and super P coated with Al 2 O 3 and Pd nanoparticles (Pd/C[Al 2 O 3 ]). The cells were discharged to a capacity of 1,000 mAh g −1 and then charged. The voltage profiles show that the charge potential is ~4.2 and ~4.4 V for the C and Al 2 O 3 -C cathodes, respectively, and that the potential is significantly reduced to about 3.2 V (compared with the theoretical 3.0 V [25] ) for the entire charge on the Pd/Al 2 O 3 /C cathode. Figure 4: Voltage profiles and SEM images. ( a ) Voltage profile during discharge-charge of cells (to 1,000 mAh g −1 ) based on super P carbon; super P carbon coated with Al 2 O 3 ; and Al 2 O 3 -coated super P carbon further coated with Pd nanoparticles. The electrolyte used is TEGDME-LiCF 3 SO 3 ; ( b ) voltage profile during discharge-charge of cells (to 5,00 mAh g −1 ) based on Al 2 O 3 -coated super P carbon further coated with Pd nanoparticles. The electrolyte used is TEGDME-LiCF 3 SO 3 . ( c ) SEM of 1st cycle after discharge to 500 mAh g −1 (scale bar, 1 μm; scale bar of inset image, 400 nm); ( d ) SEM of 1st cycle after charge, (scale bar, 1 μm); ( e ) SEM of 10th cycle after discharge to 500 mAh g −1 , (scale bar, 1 μm; scale bar of the inset image, 300 nm); ( f ) SEM of 10th cycle after charge, (scale bar, 1 μm). Full size image The observed low charge potential can be maintained for over 10 cycles at 500 mAh g −1 capacity on the Pd/C[Al 2 O 3 ] cathode as shown in Fig. 4b . After 10 cycles, the cell starts to fail with deeper discharge required and larger charge overpotentials with complete failure occurring at about 15 cycles ( Supplementary Fig. S1 ). One possible cause of the failure is the degradation of the Li anode as shown by the corrosion of the anode at termination ( Supplementary Fig. S2 ). In previous work [38] , XRD and Fourier transform infrared spectroscopic measurements have been used to analyse such corroded lithium anodes and was shown to be because of an oxygen crossover effect that results in the formation of LiOH and Li 2 CO 3 . Another possible cause of failure after 10 cycles is poisoning of the Pd catalyst by contaminants or passivation. A build-up of contaminants such as Li 2 CO 3 could be the result of gradual decomposition of the TEGDME electrolyte such as by reaction with the Li 2 O 2 surface as found experimentally [24] . We also note that when this cell is run to full discharge (2,750 mAh g −1 ), it has a much larger charge overpotential ( Supplementary Fig. S3 ). Characterization of the discharge product The discharge product was examined using SEM imaging and identified as lithium peroxide through the use of XRD. The SEM images in Fig. 4d,f show the carbon cathode after discharge and charge at the 1st and 10th cycles. The discharge product has a toroid-shaped morphology that has been found by others in Li-O 2 cells [18] , [20] , [39] . The toroids are absent from the surface of the cathode after charge as evidenced by the SEM images of Fig. 4d,f . The lithium peroxide discharge product was further probed by HRTEM imaging and results are shown in Fig. 5 . A low-magnification TEM image of a toroid is shown in Fig. 5a along with an electron diffraction pattern in Fig. 5b consistent with Li 2 O 2 . The electron diffraction pattern indicates that the toroids are nanocrystalline, which means that it consists of grains and grain boundaries. Evidence for the nanosized grains is shown in Fig. 5c . The HRTEM images in Fig. 5a also show evidence for the Pd nanoparticles in the carbon near the toroids. The XRD patterns of the discharged cathode shown in Fig. 5d demonstrate the presence of Li 2 O 2 , with no evidence of other crystalline materials such as Li 2 CO 3 or LiOH (although some trace amounts of amorphous Li 2 CO 3 or LiOH may accumulate with cycling) and the disappearance of Li 2 O 2 with charge. 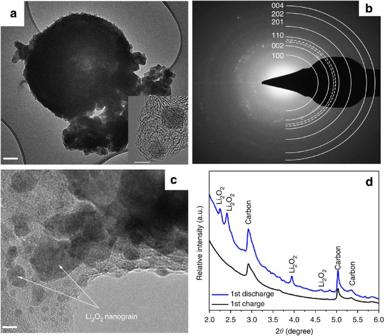Figure 5: TEM images and XRD patterns. (a) TEM image of Li2O2toroid from discharge to 2.5 V (scale bar, 100 nm), inset figure is a HRTEM image of carbon support showing the presence of Pd nanoparticles (scale bar, 3 nm); (b) electron diffraction pattern of the Li2O2toroid; (c) HRTEM image of Li2O2toroid (scale bar, 4 nm); and (d) XRD pattern of 1st discharge product showing the presence of Li2O2and the 1st cycle charge showing the absence of Li2O2on the Pd/C[Al2O3] cathode. Figure 5: TEM images and XRD patterns. ( a ) TEM image of Li 2 O 2 toroid from discharge to 2.5 V (scale bar, 100 nm), inset figure is a HRTEM image of carbon support showing the presence of Pd nanoparticles (scale bar, 3 nm); ( b ) electron diffraction pattern of the Li 2 O 2 toroid; ( c ) HRTEM image of Li 2 O 2 toroid (scale bar, 4 nm); and ( d ) XRD pattern of 1st discharge product showing the presence of Li 2 O 2 and the 1st cycle charge showing the absence of Li 2 O 2 on the Pd/C[Al 2 O 3 ] cathode. Full size image As far as we are aware, a charge overpotential as small as 0.2 V ( Fig. 4 ) has not been previously reported for a non-aqueous Li-O 2 cell. The low charge potential found here is due to a synergy of various aspects of the Pd/C[Al 2 O 3 ] cathode architecture. The effect of the Pd nanoparticles attached to the carbon surface is clearly evident from the reduction in the charge potential by about 1.2 V from the charge potential (~4.4 V) for the Al 2 O 3 -C cathode without nanoparticles in Fig. 4 . Density functional calculations in Fig. 6a show that a partially oxidized Pd nanoparticle (~1 nm) forms bonds to a defect-free graphene surface, which provides a good interface for electron transfer. This has also been noted as a key property for the use of Pd nanoparticles in sensors based on Pd nanoparticle/carbon nanotube composites [40] . In addition, the density of states of the partially oxidized Pd nanoparticle bonded to a carbon surface in Fig. 6b indicates that the Pd–C interface should be good for electronic transport across the interface needed for electrocatalysis. The electrocatalytic properties of the Pd nanoparticles are apparent from the change in the discharge potential from ~2.7 V with Pd on the cathode (Pd/C[Al 2 O 3 ]) to~2.5 V ( Fig. 4a ) when there are no Pd nanoparticles on the cathode (Al 2 O 3 /C). 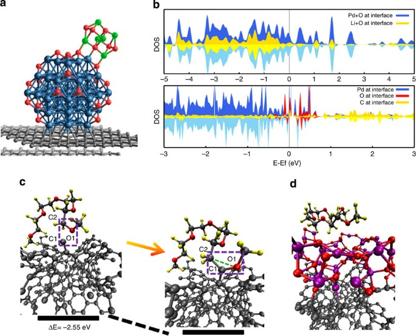Figure 6: Density functional calculations. (a) Density functional theory (DFT)-calculated structure of the Li2O2/Pd55O21/C interface, where Pd55O21represents a partially oxidized palladium nanoparticle. Colour code: palladium (blue), aluminium (purple), oxygen (red), lithium (green), hydrogen (yellow) and carbon (grey). Lithium peroxide (Li2O2) is represented by a cluster containing three Li2O2monomers. The carbon electrode (C) is represented by two stacked graphene layers. The average Pd-C bond length is 2.4 Å and the average Pd-O bond length with lithium peroxide is 2.0 Å. (b) Projected density of states at the Li2O2/Pd55O21interface (top) and Pd55O21/C interface (bottom). In both cases, only the interface atoms that are in direct contact with each other have been considered. The up and down spin electron densities are represented by dark and light colours, respectively. (c) DFT calculations of a TEGDME solvent molecule binding on a carbon defect site on a bare graphitized carbon surface. The TEGDME molecule decomposes and forms new C-O and C-H bonds on these sites. (d) Weakly bound TEDGME molecule (0.1 eV) on an Al2O3-coated carbon surface. In addition, the defect sites on the carbon-only cathode also have similar electrocatalytic properties on discharge, as the discharge potential is also ~2.7 V. Figure 6: Density functional calculations. ( a ) Density functional theory (DFT)-calculated structure of the Li 2 O 2 /Pd 55 O 21 /C interface, where Pd 55 O 21 represents a partially oxidized palladium nanoparticle. Colour code: palladium (blue), aluminium (purple), oxygen (red), lithium (green), hydrogen (yellow) and carbon (grey). Lithium peroxide (Li 2 O 2 ) is represented by a cluster containing three Li 2 O 2 monomers. The carbon electrode (C) is represented by two stacked graphene layers. The average Pd-C bond length is 2.4 Å and the average Pd-O bond length with lithium peroxide is 2.0 Å. ( b ) Projected density of states at the Li 2 O 2 /Pd 55 O 21 interface (top) and Pd 55 O 21 /C interface (bottom). In both cases, only the interface atoms that are in direct contact with each other have been considered. The up and down spin electron densities are represented by dark and light colours, respectively. ( c ) DFT calculations of a TEGDME solvent molecule binding on a carbon defect site on a bare graphitized carbon surface. The TEGDME molecule decomposes and forms new C-O and C-H bonds on these sites. ( d ) Weakly bound TEDGME molecule (0.1 eV) on an Al 2 O 3 -coated carbon surface. Full size image In addition to the electrocatalytic effect of the Pd nanoparticles, the electronic properties of the lithium peroxide discharge product resulting from the presence of the Pd nanoparticles are believed to have an important role in lowering the charge overpotential. The charge overpotential will depend on the electronic transport in the lithium peroxide discharge product [21] , [22] , [26] . As noted previously, with no limitations on electronic transport, the charge overpotential should be small. The nanocrystalline nature of the lithium peroxide discharge product for the Pd-Al 2 O 3 -C cathode ( Fig. 5 ) with small 2–10 nm grains and grain boundaries can provide a mechanism for good electronic transport for charging. This discharge product morphology may appear because the Pd nanoparticles provide nucleation sites for a form of lithium oxide growth species that assemble into the nanocrystalline Li 2 O 2 discharge product with these characteristics. We have carried out density functional calculations on amorphous lithium peroxide that is likely present in the grain boundaries, and the calculations show that amorphous Li 2 O 2 may have a metal-like density of states. ( Supplementary Fig. S4 ; the other two cathode materials (C and Al 2 O 3 /C) have much higher charge potentials (4.2–4.4 V in Fig. 4 ), which may be because of the different morphologies of the discharge products from these cathodes as shown by their s.e.m. images ( Supplementary Fig. S5 ) and also the lack of the Pd nanoparticle electrocatalyst. All the cathodes were investigated with the same TEGDME-LiCF 3 SO 3 electrolyte. It is also possible that some electrolytes have different Li 2 O 2 morphologies, which may avoid the decomposition problem. This will be the subject for a future systematic study. Finally, the Al 2 O 3 coating on the new cathode architecture also has a role in the lower charge potential found for the Pd/C[Al 2 O 3 ] Li-O 2 cell. This coating on the new cathode will prevent decomposition of the TEGDME electrolyte by blocking reaction of the TEGDME solvent molecule with the defect sites on the carbon surface. Density functional calculations were carried out on several possible types of defect sites on a graphitized surface ( Supplementary Fig. S6 ). The interaction of TEGDME with one type of carbon defect sites is shown in Fig. 6c and shows that it is exothermically very favourable to decompose by breaking a C-O bond at the site. Similar results were found at other defect sites ( Supplementary Fig. S7 ). In contrast, the density functional calculations in Fig. 6d show that an Al 2 O 3 surface is very unreactive towards the TEGDME molecule and will not result in decomposition ( Supplementary Fig. S8 ). Electrolyte decomposition on carbon defect sites will result in the deposition of contaminants such as carbonates on the lithium peroxide discharge product or on the carbon surface and likely increase the charge potential [24] . In addition, a low charge potential of <3.5 V as found for the Pd-Al 2 O 3 -C will prevent side reactions involving the carbon surface and Li 2 O 2 that may occur on charge [24] , [25] , although decomposition reactions [24] , [41] on the Li 2 O 2 surface may still occur. We also used a Li-O 2 cathode based on Pd nanoparticles (from the three cycles of ALD) on super P without the Al 2 O 3 coating. The charge potential for this cell was about 4 V ( Supplementary Fig. S9 ). This provides further evidence for the importance of a coating to passivate defect sites such as Al 2 O 3 to attain the low charge overpotentials. From the above information and the concepts in Fig. 1 , we can speculate on the mechanisms for the discharge and charge processes for the Pd/Al 2 O 3 /C cathode. If the discharge process involves electrocatalytic growth and nucleation of Li 2 O 2 nanoparticles on Pd sites, then subsequent transport through the electrolyte and aggregation could result in the nanocrystalline Li 2 O 2 morphology with small 2–10 nm grains that make up the toroids. The charge process involving decomposition of the toroids at a low charge overpotential would be facilitated by the small Li 2 O 2 grains in the toroids, conduction through grain boundaries and electronic contact with the cathode surface. In summary, a cathode architecture that utilizes nanoscale components has been shown to achieve a dramatic reduction in charge overpotential (to ~0.2 eV). The cathode promotes growth of a nanocrystalline form of lithium peroxide with electronic transport properties that are needed to lower the charge potential. In addition, the protective Al 2 O 3 coating on the cathode prevents electrolyte decomposition on carbon defect sites, which can also increase the charge potential. This new cathode architecture opens promising new avenues for Li-O 2 battery development through optimization of the metal nanoparticle and the carbon support, as well as incorporation of new protective coatings on cathodes. Cathode preparation SPL conductive carbon black with a typical particle size of 40 nm and a surface area of 62 m 2 g −1 was used as the catalyst support material. ALD was performed in a continuous-flow stainless steel reactor described in detail elsewhere. About 100 mg of the SPL carbon powder was carefully spread onto a stainless steel tray and a stainless steel mesh cover was clamped over the tray to contain the powder while still providing access to the ALD precursor vapours. The carbon powder was held in the reactor at 200 °C under continuous flow of 300 s.c.c.m. ultra-high-purity nitrogen carrier gas at 1 torr pressure for 30 min to outgas and achieve thermal equilibrium. The Al 2 O 3 ALD used alternating exposures to trimethylaluminium (Sigma-Aldrich, 97%) and deionized water at 200 °C. Exposure/purge time 60 -120-60-180 s was used. The three cycles of Al 2 O 3 ALD on the carbon black powder were performed to cover the carbon defect sites. After the Al 2 O 3 ALD cycles, the Pd ALD was then performed using alternating exposures to palladium hexafluoroacetylacetonate (Pd(hfac) 2 , Aldrich, 99.9%) and formalin (Sigma-Aldrich, HCHO 37 wt% in H 2 O) at 200 °C. Timing sequence of a complete ALD cycle can be expressed as t 1 - t 2 - t 3 - t 4 , corresponding to the precursor exposure time, N 2 purge time, co-reactant exposure time and N 2 purge time, respectively. The timing sequence utilized for the Pd ALD was 100-300-100-300. Catalyst samples were prepared using three Pd ALD cycles on the three cycles of ALD AL 2 O 3 -coated carbon powder. Electrochemical methods Electrochemical characterization was carried out using a Swagelok-type cell composed of a lithium metal anode, electrolyte (1 M LiCF 3 SO 3 in TEGDME impregnated into a glass fibre separator) and a porous cathode (13 mm diameter). The cathode was formed by casting a mixture of the as-prepared Pd/SPL carbon and binder in a molar ratio of 80:20. The cells were sealed except for the Al grid window that exposed the porous cathode to 1 bar O 2 pressure. The electrochemical measurements were carried out using a Biologic MacPile cycler. The discharge-charge performance was conducted in at a constant current of 100 mA g −1 , and the cell was maintained in 1 bar O 2 atmosphere to avoid any negative effects of humidity and CO 2 . For comparison, a blank SPL carbon without any catalyst was also tested using the same cell configuration described above. We normalized the observed capacity by the weight of the carbon and catalyst for comparison in this study. X-ray absorption spectroscopy Pd K-edge (23.564 keV) XAS was performed at the Materials Research Collaborative Access Team at the Advanced Photon Source, Argonne National Laboratory. The sample was loaded as a self-supporting wafer without binder in the channels (internal diameter, 4 mm) of a stainless steel multisample holder. The sample holder was then placed in the centre of a quartz tube, which was equipped with gas and thermocouple ports and Kapton windows. The amount of sample used was optimized to achieve an XAS step height of about 0.5. The XAS spectra were recorded in transmission mode. The Pd fraction was calculated by conducting Pd XANES linear combination fittings using Athena in the IFEFFIT (version 1.2.11) package. XANES reference spectra were collected using a metallic Pd foil and a Pd oxide sample. Standard procedures based on WINXAS 3.1 software were used to fit the data in the extended X-ray abosrption fine structure regime. The extended X-ray abosrption fine structure coordination parameters were obtained by a least-square fit in q- and r-space of the isolated nearest neighbour, k 2 -weighted Fourier transform data. High-energy XRD The cathode laminates after discharge were characterized by high-energy synchrotron XRD to determine the formation of Li 2 O 2 , which was carried out at the 11-ID-C beamline of the Advanced Photon Source, Argonne National Laboratory. The X-ray wavelength was 0.10804 Å. The samples were completely covered with Kapton tape as a protective film in the glove box to avoid any side reactions from the air. The XRD patterns were collected in the transmission mode using a Perkin Elmer large area detector. The collected two-dimensional patterns were then integrated into conventional one-dimensional patterns (intensity versus 2 θ ) for final data analysis using the Fit2d software. X-ray photoelectron spectroscopy Samples were analysed by XPS using a Kratos Axis Ultra DLD surface analysis instrument. The base pressure of the analysis chamber during these experiments was 3 × 10 −10 torr, with operating pressures around 1 × 10 −9 torr. Spectra were collected with a monochromatic Al Kα source (1486.7 eV) and a 300 μ × 700 μ spot size. Before introduction into the load-lock vacuum chamber of the XPS instrument, all air-sensitive samples were loaded into an inert transfer module interfaced with the instrument. Samples were prepared in an Ar-filled glove box, with no more than 1 p.p.m. O 2 and 1 p.p.m. H 2 O. Non-conductive samples showed evidence of differential charging, resulting in peak shifts and broadening. Photoelectron peak positions were shifted back towards their true values and their peak widths were minimized by flooding the samples with low-energy electrons and ions from the charge neutralizer system on the instrument. Peak position correction was further corrected by referencing the C 1s peak position of adventitious carbon for a sample (284.8 eV, PHI Handbook of Photoelectron Spectroscopy) and shifting all other peaks in the spectrum accordingly. Fitting was done using the program CasaXPS. Peaks were fit as asymmetric Gaussian/Lorentzians, with 0–30% Lorentzian character. The FWHM of all sub-peaks was constrained to 0.7–2.0 eV, as dictated by instrumental parameters, lifetime broadening factors and broadening due to sample charging. With this native resolution set, peaks were added and the best fit, using a least-squares fitting routine, was obtained while adhering to the constraints mentioned above. Electron microscopy A field-emission transmission electron microscope with a spherical and chromatic aberration imaging corrector working at 80 kV was employed to evaluate the morphology and particle size of the ALD Pd catalysts, Al 2 O 3 and Li 2 O 2 toroids. Operation at 80 kV was used to avoid knockout damage to carbon materials from the electron beam. Spherical and chromatic aberration correction enables the microscope to attain resolution better than 0.1 nm (measured by Young’s fringes) at 80 kV. To prepare the TEM specimens, holey carbon grids were placed in the bottle of as-received powders and shaken to allow small powders to attach on the holey carbon. No liquid was used to avoid possible morphology change owing to the interaction with solution. Theoretical calculations All the density functional theory simulations (that is, geometry optimizations and energy calculations) were carried out based on plane wave basis functions. All the calculations were spin-polarized and carried out using the gradient-corrected exchange-correlation functional of Perdew, Burke and Ernzerhof. For the amorphous graphitized carbon slab (with total 264 atom), the initial amorphous geometry was obtained from classical many-body molecular dynamic simulation followed by full geometry relaxation using density functional theory. The oxidized palladium nanoparticle was represented by a Pd 55 O 21 cluster with ~1 nm particle size and cuboctahedron shape with the oxygen atoms occupying the hcp hollow positions of the available palladium (111) facets. The stacked two-layer graphene consists of 256 carbon atoms (with the bottom layer kept fixed during relaxation). For the amorphous Li 2 O 2 bulk structure used to model the grain boundaries, the optimized geometry was obtained by randomly placing 54 Li 2 O 2 molecules inside a cubic simulation cell (12 Å × 12 Å × 12 Å) after simulated annealing and lattice cell relaxation. More details can be found in Supplementary Methods . How to cite this article: Lu, J. et al. A nanostructured cathode architecture for low charge overpotential in lithium-oxygen batteries. Nat. Commun. 4:2383 doi: 10.1038/ncomms3383 (2013).